Discrete plasticity in sub-10-nm-sized gold crystals Although deformation processes in submicron-sized metallic crystals are well documented, the direct observation of deformation mechanisms in crystals with dimensions below the sub-10-nm range is currently lacking. Here, through in situ high-resolution transmission electron microscopy (HRTEM) observations, we show that (1) in sharp contrast to what happens in bulk materials, in which plasticity is mediated by dislocation emission from Frank-Read sources and multiplication, partial dislocations emitted from free surfaces dominate the deformation of gold (Au) nanocrystals; (2) the crystallographic orientation (Schmid factor) is not the only factor in determining the deformation mechanism of nanometre-sized Au; and (3) the Au nanocrystal exhibits a phase transformation from a face-centered cubic to a body-centered tetragonal structure after failure. These findings provide direct experimental evidence for the vast amount of theoretical modelling on the deformation mechanisms of nanomaterials that have appeared in recent years. Plastic deformation in micro- and sub-micrometre metallic crystals is well documented [1] , [2] , [3] . However, the deformation mechanisms of sub-10-nm-sized crystals remain unclear [4] , [5] , [6] , [7] , [8] , [9] , [10] , [11] , [12] . It has been widely accepted that the sample size may exert significant influence on the mechanical, electrical, optical and magnetic properties of nanomaterials. Recently, direct experimental observations of source-controlled dislocation plasticity in sub-micrometre aluminium single crystals [13] were reported. At this length scale, single-ended dislocation sources are predominantly active with much smaller source lengths compared with double-pinned Frank-Read sources. The authors point out that the balance between the dislocation nucleation rate and loss rate is responsible for the flow stress. A natural question that arises is: how do materials behave when dislocation ensembles are not present? Specifically, what are the controlling factors that determine the flow stress of nanometre-sized metals? As sample dimensions decreases down to the nanometre scale, where Frank-Read-like sources should no longer be active, plasticity should be surface dominated; however, the location of dislocation nucleation sites and the mechanisms by which the dislocations nucleate are still unclear [5] , [7] , [9] . When the crystal size reaches atomic dimensions, the strength of the material is governed by the bond strength of atomic chains [14] , [15] , [16] . However, to the best of our knowledge, there is a lack of experimental evidence regarding the deformation mechanisms in sub-10-nm-sized crystals because of the difficulty in handling these small crystals, although they are reported to be ultrastrong compared with their bulk counterpart, as predicted from both theoretical calculations [17] and experimental observations [10] , [12] . So far, our understanding of the deformation behaviour of metallic nano-sized crystals relies heavily on molecular dynamics (MD) simulations, which may suffer from the accuracy of empirical or semi-empirical inter-atomic potentials and high strain rates. Although MD predictions offer insight into the deformation behaviour of nanocrystals, it is still debatable whether or not these simulation results can be directly extrapolated to laboratory conditions. For example, a number of MD simulations have revealed dislocation activity in single metallic nanocrystals during both tension [4] , [5] , [6] , [11] and compression tests [5] , [6] , [9] , and it is argued that the plastic deformation in nanocrystals is dominated by short-lived dislocations, which may not be examined by the available experimental techniques [10] . Therefore, new experimental studies are needed to validate some predicting results from MD simulations [4] , [5] , [6] , [9] . In this study, we employ an in situ tensile testing technique using high-resolution transmission electron microscopy (HRTEM) to reveal the deformation process in nanometre-sized face-centered cubic (FCC) Au. In this work we show that (1) partial dislocations that nucleate from the free surface dominate the plastic deformation; (2) in addition to the crystallographic orientation (Schmid factor), the character of the free surfaces may have a non-negligible role in determining the deformation mechanism; and (3) after unloading, surface stresses can induce phase transformations in nanocrystals. 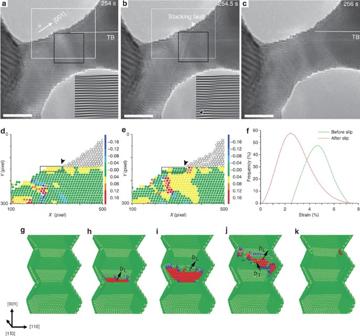Figure 1: Tensile loading test of an Au nanocrystal. This tensile test (see alsoSupplementary Movie 1) shows that surface steps act as the dislocation sources (see alsoSupplementary Movie 2). (a–c) Sequential HRTEM images showing the emission of a dislocation from a free surface. The insets ina,bFourier-filtered images (reconstructed using the spatial frequencies of the (111) planes) of the black square area, respectively. The scale bar in each figure represents 3 nm. (d,e) The strain mapping of the white-boxed area in HRTEM images beforeaand afterbshows the nucleation of a partial dislocation. The black arrowheads indicate the site for dislocation nucleation. Open circles on the upper right part of the two figures represent the twinning lamella. (f) A quantitative strain analysis of the black-boxed region indande; frequency is the number of atoms with that strain divided by the total number of atoms in the black-boxed area indande. (g–k) MD simulations illustrating the atomic process of nucleation (h), propagation of the leading partial producing a stacking fault (i) and the nucleation of the trailing partial (j), wherebLandbTmark the location of leading and trailing partials, respectively. Eventually, the combined perfect dislocation leaves out of the sample (k). Colours are assigned to the atoms according to a local crystallinity classification visualized by common neighbour analysis (see Methods for details). Surface-mediated plastic deformation Figure 1 shows the tensile loading of an Au nanocrystal under a strain rate of 10 −3 s −1 . The beam is orientated along the [11̄0] and the tensile loading direction is [001] ( Fig. 1a ). Figure 1a shows an abundance of {111} facets, which have the lowest surface energy, separated by surface steps on the Au crystal surface. It should be noted that the {111} facets are also frequently encountered in as-synthesized FCC nanocrystals [18] . Interestingly, a pre-existing twin boundary is present as well. On tensile loading, dislocation emission from the grain boundary near the left contact was observed ( Supplementary Figs S1 and S2 , Supplementary Movie 1 and Supplementary Discussion ). Figure 1: Tensile loading test of an Au nanocrystal. This tensile test (see also Supplementary Movie 1 ) shows that surface steps act as the dislocation sources (see also Supplementary Movie 2 ). ( a – c ) Sequential HRTEM images showing the emission of a dislocation from a free surface. The insets in a , b Fourier-filtered images (reconstructed using the spatial frequencies of the (111) planes) of the black square area, respectively. The scale bar in each figure represents 3 nm. ( d , e ) The strain mapping of the white-boxed area in HRTEM images before a and after b shows the nucleation of a partial dislocation. The black arrowheads indicate the site for dislocation nucleation. Open circles on the upper right part of the two figures represent the twinning lamella. ( f ) A quantitative strain analysis of the black-boxed region in d and e ; frequency is the number of atoms with that strain divided by the total number of atoms in the black-boxed area in d and e . ( g – k ) MD simulations illustrating the atomic process of nucleation ( h ), propagation of the leading partial producing a stacking fault ( i ) and the nucleation of the trailing partial ( j ), where b L and b T mark the location of leading and trailing partials, respectively. Eventually, the combined perfect dislocation leaves out of the sample ( k ). Colours are assigned to the atoms according to a local crystallinity classification visualized by common neighbour analysis (see Methods for details). Full size image On further tensile loading, the grain boundary ceases to be a source for dislocations and the surface steps enlarge through slip in order to accommodate the tensile deformation ( Fig. 1 ). These steps are located at the intersection of two sets of {111} planes and serve as dislocation nucleation sources. Figure 1a–c consists of sequential HRTEM images showing the entire process of dislocation dynamics involving the nucleation of a leading partial from a surface step ( Fig. 1a ), the stacking fault (as pointed out by an arrowhead in the inset of Fig. 1b ) and the trailing partial, which eliminates the stacking fault ( Fig. 1c ; see Supplementary Movie 2 . For clarity, the identification of different dislocation types on the basis of the HRTEM images is illustrated as well ( Supplementary Figs S3–S5 )). Our experimental results illustrate for the first time that surface steps can serve as dislocation sources to accommodate plastic deformation of metallic nanocrystals. To further understand the mechanics of partial dislocation emission from free surfaces, a quantitative lattice strain analysis was performed using lattice distortion analysis (LADIA) [19] on the HRTEM images acquired before ( Fig. 1a ) and after ( Fig. 1b ) the leading partial was nucleated. The lattice strain distribution along [001] loading direction of the white-boxed area in Figure 1a,b are shown in Figure 1d,e , respectively. The localized stress concentration near the surface step [20] is directly visualized in Figure 1d (indicated by the black arrow head). A quantitative strain profile ( Fig. 1f ) of the surface area enclosed by black boxes (used as lattice strain gage) in Figure 1d,e indicates that the mean elastic strain is 0.048 and 0.028, before and after partial dislocation nucleation, respectively. Assuming that slip occurred through a partial dislocation on a 〈112〉{111} slip system, the resolved shear stress for the dislocation nucleation is estimated to be 0.47 GPa (given that the Young's modulus is 42 GPa [21] along the [001] and the Schmid factor is 0.23), which drops after partial dislocation emission from the surface (the error estimation is discussed in the Methods section, see also Supplementary Fig. S6 ). Figure 1g–k shows snapshots of dislocation nucleation in a nanocrystal dominated by {111} facets, as modelled by MD simulations. The simulation methodology and associated details can be found in the Methods section. A leading partial nucleates from a surface step (marked by a letter ' b L ' in Fig. 1h ), propagates on a {111} slip plane leaving behind a stacking fault ( Fig. 1i ), which is followed by the trailing partial dislocation (marked by a letter ' b T ' in Fig. 1j ) that eliminates the stacking fault. The simulation result is consistent with our experimental observations ( Fig. 1a–c ) in that the surface steps are sites for dislocation nucleation and that, in the presence of these facets, the dominant mechanism of plastic deformation is through partial dislocation slip involving both leading and trailing partial dislocations. Discrete necking process With extensive tensile elongation, necking occurs in the nanocrystal ( Fig. 2 ), which is a result of discrete cooperative slip events on two conjugate {111} planes, giving rise to a number of enlarged surface steps ( Fig. 2a–c , see also Supplementary Movie 3 ). The surface steps are one or two atomic planes apart, exhibiting a saw-tooth morphology. These discrete surface steps could correspond to the quantized plastic deformation observed in tensile-deformed Au nanowires (NWs) conducted by atomic force microscope, wherein the length of the NW was characterized by quantized increment due to the slippage between {111} planes [22] . 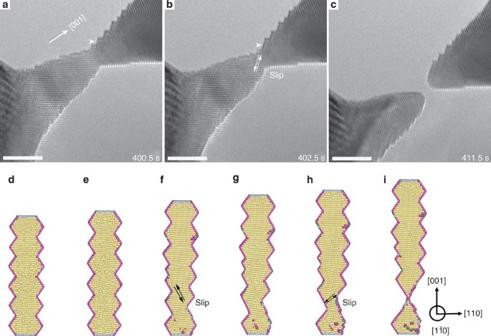Figure 2: Necking of the nanocrystal. The figure depicts the same nanocrystal shown inFigure 1(see alsoSupplementary Movie 3). (a,b) The experimental observations of the cooperative slip between two conjugate {111} planes, leading to the enlargement of the surface steps indicated by the arrowheads. A 10% elastic strain is estimated from the change of the (002) lattice plane spacing. (c) Final fracture of the nanocrystal. The scale bar in each figure represents 3 nm. (d–i) A profile view of the MD simulations of the necking process induced by slip. Atoms are coloured according to the coordination numbers (seeSupplementary Materialsfor details). The necking process induced by slip in Figure 2a,b is also clearly captured in our MD simulations ( Fig. 2d–i ). Figure 2f,h specifically shows slip along two sets of {111} planes. When the inhomogeneous deformation occurs in MD simulations, relative slip between two adjacent {111} planes is accompanied by rapid cross-section area reduction, similar to Figure 2a,b . One noticeable difference is the final fracture surface. Fracture in experiments shows a {001} surface enclosed by {111} facets, whereas MD simulations only show {111} facets. The differences could be caused by a number of factors including the stiffness of the loading frame, strain rate effects of MD simulations or the assumed geometry in the MD model. Figure 2: Necking of the nanocrystal. The figure depicts the same nanocrystal shown in Figure 1 (see also Supplementary Movie 3 ). ( a , b ) The experimental observations of the cooperative slip between two conjugate {111} planes, leading to the enlargement of the surface steps indicated by the arrowheads. A 10% elastic strain is estimated from the change of the (002) lattice plane spacing. ( c ) Final fracture of the nanocrystal. The scale bar in each figure represents 3 nm. ( d – i ) A profile view of the MD simulations of the necking process induced by slip. Atoms are coloured according to the coordination numbers (see Supplementary Materials for details). Full size image Phase transition from FCC to BCT After fracture, the crystal unloads and, in some cases, undergoes a phase transformation from a FCC to body-centered tetragonal (BCT) structure ( Fig. 3 ), which is predicted in recent theoretical work by Diao et al . [23] It is theorized that the transformation occurs when compressive stresses caused by the tensile surface stress components along the 〈001〉 direction exceed the stress required to transform bulk gold (Au; FCC) to its higher-energy crystal structure (BCT). Our experimental observation provides the first direct evidence of such kind of phase transformation. 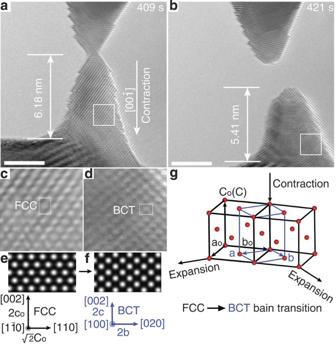Figure 3: Surface stress-induced phase transformation. (a) The moment before nanocrystal fractures. (b) The contraction (relaxation) of the bottom part of Au crystal after the crystal fractures. The scale bar in each figure represents 3 nm. (c,d) Enlarged HRTEM images of the white-boxed area inaandb, respectively, accompanied with the corresponding crystallographic orientation. (e) Simulated HRTEM image of FCC Au along [110] zone axis with lattice parameter ofa=4.078 Å. (f) Simulated image of BCT Au along [100] zone axis with lattice parameter ofa=b=3.34 Å andc=2.86 Å. The simulations were conducted by applying the parameters including the acceleration voltage of 300 kV, spherical aberration coefficient of the 1.2 mm, the specimen thickness of 3 nm and the focus value of −43 nm. (g) Martensitic transition (FCC–BCT) due to lattice distortion along [001] direction in FCC crystal on the basis of the Bain path. The unit cells of FCC and BCT crystals are outlined with black and blue lines, respectively. As can be clearly seen in Figure 3a,b (see also Supplementary Movie 3 ), the bottom half of the nanocrystal contracts after fracture. The HRTEM images indicating the transformation from FCC to BCT is shown in Figure 3c,d . The lattice constants of FCC are a o = b o = c o =4.07 Å, whereas those of BCT phase are determined to be a = b =3.34 Å and c =2.86 Å (the error estimation is presented in the Methods section, see also Supplementary Fig. S7 ). Correspondingly, a lattice contraction of 30% along the length direction (〈001〉 direction) is obtained, in accordance with the theoretical prediction [23] . In addition, the phase transition can be well explained by the Bain model [24] , which suggests that on biaxial expansion of the lattice constant in the {001} plane, a FCC solid may transform spontaneously into a body-centered cubic or BCT phase through relaxation of the interlayer spacing along the perpendicular 〈001〉 direction ( Fig. 3g ). It is worth noting that the theory has also predicted that Au nanocrystals may re-orient to 〈110〉 FCC crystals rather than transforming to BCT [25] . However, the lattice image in Figure 3d cannot be interpreted according to a FCC Au structure, which rules out the possibility of reorientation mechanism that was proposed [25] . Additionally, the simulated images of a FCC Au crystal along [110] zone axis ( Fig. 3e ) and a BCT Au crystal along the [100] zone axis ( Fig. 3f ) agree with the experimental observed HRTEM images shown in Figure 3c,d, respectively. In our experiment, the phase transformation is only observed in the fractured, or relaxed, nanocrystal after 〈001〉 tensile loading, consistent with the MD simulation results. As the compressive stresses induced in the core of the nanocrystal by the surface stress scale inversely with the size of the crystal, phase transformation is a size-dependent phenomenon. Our experiments show that the top half remains FCC ( Fig. 3b ), which may result from the crystal being larger or different surface stresses as a result of faceting. From MD predictions, the transformation was observed in 2.65 nm×2.65 nm NW with cross-sectional area of 7 nm 2 (at room temperature 300 K) [23] , which we believe is quite close to that of the nanocrystal observed in the current experiment ( Fig. 3b ). Figure 3: Surface stress-induced phase transformation. ( a ) The moment before nanocrystal fractures. ( b ) The contraction (relaxation) of the bottom part of Au crystal after the crystal fractures. The scale bar in each figure represents 3 nm. ( c , d ) Enlarged HRTEM images of the white-boxed area in a and b , respectively, accompanied with the corresponding crystallographic orientation. ( e ) Simulated HRTEM image of FCC Au along [110] zone axis with lattice parameter of a =4.078 Å. ( f ) Simulated image of BCT Au along [100] zone axis with lattice parameter of a = b =3.34 Å and c =2.86 Å. The simulations were conducted by applying the parameters including the acceleration voltage of 300 kV, spherical aberration coefficient of the 1.2 mm, the specimen thickness of 3 nm and the focus value of −43 nm. ( g ) Martensitic transition (FCC–BCT) due to lattice distortion along [001] direction in FCC crystal on the basis of the Bain path. The unit cells of FCC and BCT crystals are outlined with black and blue lines, respectively. Full size image Tensile loading of nanocrystals along different directions We also found that the tensile loading direction affects the deformation mechanisms of sub-10-nm Au significantly. 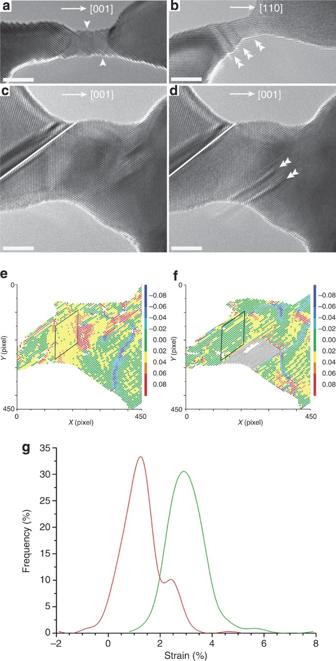Figure 4: Dislocation slip and deformation twinning with their quantitative strain analysis. (a,b) Ina, individual slip dominates the plastic deformation for a [001] loading, whereas inbtwinning is the main deformation mode for [110] loading, see alsoSupplementary Movies 1,2and3. (c,d) Sequential images captured before and after the twinning partials are emitted; the double arrowheads indicate the location of the deformation twins. The scale bar in each figure represents 4 nm. (e,f) The strain mapping of the HRTEM images ofcandd, respectively, showing a strain relaxation immediately after the twin formation. Likewise, the open circles are drawn to represent the twinning partials. (g) A quantitative strain analysis, performed using the LADIA software, of the black-box region ineandf, showing data before (green curve) and after twinning (red curve). All images are taken along the [11̄0] zone axis. The surface steps indicated by the arrowheads are caused by partial dislocation slip and the double arrowheads show the deformation twins. Figure 4a,b (see Supplementary Movies 4 and 5 ) shows that slip and twinning are favoured under 〈001〉 and 〈110〉 tensile loading directions, respectively, which confirms theoretical predictions [5] . The dominant effect is the Schmid law, which indicates that the slip system with highest Schmid factor is preferred on the deformation modes in small-scale materials. For the 〈001〉 orientation, the Schmid factor for the trailing partial is higher than the leading partial, which suggests that slip is preferred. However, for the 〈110〉 direction, the Schmid factor for leading partial is higher, which therefore enhances the propensity of twinning [5] . Figure 4: Dislocation slip and deformation twinning with their quantitative strain analysis. ( a , b ) In a , individual slip dominates the plastic deformation for a [001] loading, whereas in b twinning is the main deformation mode for [110] loading, see also Supplementary Movies 1 , 2 and 3 . ( c , d ) Sequential images captured before and after the twinning partials are emitted; the double arrowheads indicate the location of the deformation twins. The scale bar in each figure represents 4 nm. ( e , f ) The strain mapping of the HRTEM images of c and d , respectively, showing a strain relaxation immediately after the twin formation. Likewise, the open circles are drawn to represent the twinning partials. ( g ) A quantitative strain analysis, performed using the LADIA software, of the black-box region in e and f , showing data before (green curve) and after twinning (red curve). All images are taken along the [11̄0] zone axis. The surface steps indicated by the arrowheads are caused by partial dislocation slip and the double arrowheads show the deformation twins. Full size image Our in situ observations also show that the deformation mechanism of Au nanocrystals may change from dislocation slip ( Fig. 4a ) to twinning ( Fig. 4c,d ; see Supplementary Movie 6 ) under the same 〈001〉 loading direction. MD predictions have shown a transition from slip to twinning as a function of the NW aspect ratio [26] ; however, as our images are two-dimensional, aspect ratios cannot be determined. Figure 4a shows the abundance of {111} terraces, where the slip occurs. Slip from these surface facets is most likely favoured because slip enlarges the {111} facets already present, which are the lowest energy surfaces. It is worth noting that the twinning partials shown in Figure 4b,d apparently nucleate from the free surface, illustrating again that the surfaces serve as sources for the plastic deformation. Lattice strain analysis with the LADIA software has been performed on the HRTEM images acquired before ( Fig. 4c ) and after ( Fig. 4d ) the nucleation of twinning partials. The lattice strain distribution along [001] loading direction of the right side of the white lines in Figure 4c,d are shown in Figure 4e,f , respectively. A quantitative strain profile ( Fig. 4g ) of the black-boxed area (used as lattice strain gage) in Figure 4e,f indicates that in before and after twin formation, the mean elastic strain is 0.030 and 0.013, respectively. From the strain analysis, a tensile stress of 1.28 GPa (corresponding to 0.29 GPa of shear stress) is estimated for the nucleation of the twinning partials, whereas after twinning the tensile stress is relieved to 0.53 GPa. As the stresses for dislocation and twin nucleation should be sensitive to surface conditions, we have characterized the surfaces in Figures 1a and 4c (as shown in Supplementary Figs S8 and S9 , respectively). Electron beam effects were major factors in our search for the appropriate material to use in these tensile loading experiments. There are two major electron beam effects, both of which are negligible in our experiment. (1) Knock-on displacement : if the energy of the electron beam exceeds the displacement threshold energy E d , which is material dependent (bond strength, crystal lattice and atomic weight of the constituent atoms), then high-angle elastic scattering can displace atomic nuclei to interstitial positions, thereby degrading the quality of the crystal. However, to create such damage in Au, a threshold energy of 1,320 KeV is needed [27] . Thus, the 300 KV acceleration voltage applied in our experiments is too low to produce such kind of beam damage. Although the surface displacements of Au atoms might be possible, its influence on the plastic deformation behaviour might be small [28] . (2) Beam heating : first, Au is a material with high thermal conductivity (300 W mK −1 ) and is therefore able to conduct heat away quickly. Following the discussion by Williams [28] , it is unlikely that the radiation will be a significant factor unless the thermal contact is very poor. Therefore, beam heating is not significant as the Au nanocrystals are welded to a Au thin film whose size is much larger compared with the volume of the sample. Although the beam current applied to get the HRTEM images of dislocation dynamics in these Au nanocrystals ranged from 80 to 100 A cm −2 , we believe that the temperature rise is not significant [29] . Finally, such small temperature rises would have little effects on dislocation nucleation [7] . There have been many predictions regarding the plastic deformation of NWs using MD simulations [4] , [5] , [6] , [7] , [9] , [11] , [16] , [17] , [26] ; however, a major criticism of this approach is the associated high strain rates. These experiments show that plastic deformation in 〈100〉 oriented Au nanocrystals is dominated by leading and trailing partials, whereas in the 〈110〉 oriented nanocrystal, twinning is frequently observed. Our MD simulations show that slip occurs through leading and trailing partials for 〈100〉 oriented crystals in the presence of {111} surface facets, in agreement with our experiments. These experimental results are also in general agreement with Park et al . [5] who predicted that slip should dominate the tensile deformation of 〈100〉 NWs and twinning in tensile deformation of 〈110〉 wires. Our results disagree with the specific prediction of Liang et al . [6] , who show that the tensile deformation of 〈100〉 wires should be through the propagation of partial dislocations only, as our observations show that the trailing partial dislocation is also involved. The experiments do confirm that MD simulations are useful in understanding plasticity in metallic NWs, despite the differences in strain rates. The discrepancy with Liang et al . [6] is likely due to the use of pristine square geometries, which are not realized in experiments and is another confirmation of the importance of surface facets on the deformation of NWs [5] , [26] and highlights the usefulness of a combined experimental and modelling approach. Furthermore, because of the influence of the geometry on deformation, it is not yet possible to make direct comparisons of strength with existing simulations of engineered structures [17] , and further experimental investigation is warranted. In summary, the present in situ HRTEM tensile loading investigation highlights the distinct differences in the plastic deformation mechanisms between sub-micrometre- and nanometre-sized single crystals. In the former, plasticity is controlled by single-armed sources, whereas in the latter the plasticity is surface dominated. It confirms three key things that have been predicted by theory and simulation. First, discrete plastic deformation events (individual slip) from surfaces are directly observed and their dynamics and nucleation stresses are revealed through in situ HRTEM images and the corresponding lattice strain analysis. The stress concentration in the vicinity of surface steps is directly captured in our experiment, making the surface steps the preferential sites for dislocation nucleation. Second, additionally, the deformation mechanism of nanometre-sized Au is not determined by purely crystallographic orientation (Schmid factor) and likely depends on the character of the free surfaces. Third, it is shown that after unloading, surface stresses can cause phase transformations in Au nanocrystals, which is size dependent and a property unique to nanoscale materials. Our experiments show, in general, that MD simulations are useful despite the large differences in strain rates. Additionally, our results directly confirm that plasticity is still mediated by dislocations, removing the possibility of diffusional creep, which may be overlooked by MD simulations. Finally, MD simulations have also shown that the free surface facets have a significant role in influencing plasticity [5] , [26] , which is again consistent with our direct in situ observations. Sample preparation and experimental methods Our experiments were conducted inside a FEI Tecnai F30 field emission gun transmission electron microscope (TEM) equipped with a Nanofactory TEM-STM system [30] . The TEM was operated at 300 kV, with a point-to-point resolution around 0.2 nm. The videos containing dislocation dynamics were recorded by a CCD (charge-coupled device) camera at 2 frames per s. The Au NWs and NPs were prepared by reducing AuCl (oleylamine) complex with 10-nm Ag NPs in hexane. Briefly, 10-nm Ag NPs were first synthesized by decomposing 0.22 g silver trifluoroacetate in 10 ml isoamyl ether and 0.66 ml oleylamine at 160 °C for 1 h under the protection of argon gas. The Au NWs and NPs were obtained by mixing 10 mg AuCl and 0.28 ml oleylamine in 2.15 ml of hexane, heated to 60 °C and then reacted with 0.05 ml of the as-prepared, 10-nm Ag NPs at 60 °C for 45 h. For details, please refer to the previous publication [31] . First, the Au NWs and NPs were attached to a piezo-operated scanning tunnelling microscope (STM) probe with silver paint, which served as one end of a Nanofactory TEM-STM platform. A wedge-shaped Au wafer was the other end of platform. Second, the STM probe with the Au crystals on its tip was compressed onto an Au thin foil substrate. During the compression process, the Au crystals on the STM tips were cold welded [32] to the Au substrate, forming a strong contact. Third, the STM probes were retracted from the Au substrate ( Supplementary Fig. S10 ). During the retraction of the STM probe, the Au crystals between the Au substrate and the STM tip underwent tensile deformation. MD simulation details The MD simulations of the tensile elongation of Au nanocrystals were carried out using LAMMPS package [33] . The velocity-Verlet integrator with time step of 2 fs was used in the entire simulations. The embedded atom method potential [34] was used to model the Au inter-atomic interactions. Before mechanical loading, energy minimization was performed by means of the conjugate gradient method to relax the structure. Free surface boundary conditions were used in all three dimensions. The nanocrystals were then thermally equilibrated to 300 K for 20 ps using a Nosé–Hoover thermostat. Starting from the equilibrium configuration of the nanocrystals, uniaxial tensile loading was applied until failure. During the tensile loading process, the clamped upper end, consisting of two layers of atoms, was continuously pulled at a constant velocity of 0.01 Å ps −1 along the loading direction. The resulting strain rate was 6×10 7 s −1 . To discern defects in the NWs, colours are assigned to the atoms according to a local crystallinity classification visualized by common neighbour analysis, which permits the distinction between atoms in a local hexagonal close-packed (HCP) environment and those in a FCC environment. Perfect FCC atoms are removed for clarity, red stands for HCP atoms, green for other 12 coordinated atoms and blue for the non-12-coordinated atoms. A single line of HCP atoms represents a twin boundary; two adjacent HCP lines stand for an intrinsic stacking fault. Other 12 coordinated atoms and non-12-coordinated atoms appear in the free surface region and in the core of dislocations. Error estimation The error of estimating the lattice strain by employing the LADIA software is evaluated as follows: lattice distortion analysis was performed on an experimental micrograph taken from a distortion-free Au NW object viewed in the 〈110〉 projection ( Supplementary Fig. S6a ). The normal strain along the 〈001〉 direction was measured ( Supplementary Fig. S6b ) within a selected area in the micrograph (white box in Supplementary Fig. S6a ), which is similar to those for the measurements presented in this work. The deviation of the strain values measured for different image peaks is not due to the structure of the material, but to the noise in the micrograph and to the limit of the peak position measurement. Twice the measured deviation (±0.008) reveals the detection limit [35] of the analysis method for individual image peak. This represents the majority of the error in the lattice distortion analysis. For Figure 1d,e , as the histogram was extracted from the strain gage at the edge of the specimen, the effect of local thickness variation should be negligible. Meanwhile, a possible twist or rotation of the NW, which will cause local misorientation of the crystal, will not introduce notable errors to the results of Figure 1f , also due to the very thin sample edge. We find that the image feature and image contrast are constant through the in situ experiment, which suggest that either the focus setting or the height of the specimen remains the same during the whole experiment. These make the comparison of the averaged strains determined from the strain gages in Figure 1a,b reliable. For Figure 4e,f , before and after the twinning formation, the thickness of the specimen along the viewing direction should remain the same. Meanwhile, the image feature and image contrast remain constant in the strain gage region. As examined by our previous image simulations [36] , slight bending or twisting of the NW will not have a notable influence on the measurement. The strain values used for the calculation of stress release of twinning formation were determined from the averaged strain in the gage; therefore, the local thickness variation or misorientation should not influence the averaged values. The lattice constants of FCC and BCT crystals are directly measured. Repeated measurements in different areas reveal that the standard deviation lattice constant of the FCC and BCT phase is 0.04 Å ( Supplementary Fig. S7a ) and 0.03 Å, respectively ( Supplementary Fig. S7b ). Characterization of surfaces in Figures 1a and 4c As the stresses for dislocation and twin nucleation should be sensitive to surface conditions, we have characterized the surfaces in Figures 1a and 4c . There are many surface steps enclosed by {111} planes, as shown in Figure 1a , including two types of surface steps: single atomic height step (similar to step 2 shown in Supplementary Fig. S5 ) and double atomic height step (similar to step 3 shown in Supplementary Fig. S5 ). If we restrict our analysis to the crystal length (9.52 nm) between the two white lines shown in Supplementary Figure S8a , the length density of single atomic height steps (hereafter called 'single steps') and double atomic height steps (hereafter named as 'double steps') are calculated to be 0.53 nm −1 and 0.37 nm −1 , respectively. It is interesting to note that the nucleation occurs more on the upper surface, where more steps (regardless of the step height) are present, compared with the bottom surface of the nanocrystal. The average terrace width is 1.2 nm. The structure and surface dilation is estimated by measuring the distance between two neighbouring atoms along the [1̄1̄2] direction. We obtain an average value of 2.66 Å for the region near the dislocation nucleation site (enclosed area in Supplementary Fig. S8b ) and 2.53 Å for surface area outside of the white box ( Supplementary Fig. S8c ). Compared with the average value (2.53 Å) inside the crystal ( Supplementary Fig. S8d ), a lattice dilation of 5% is estimated in the surface dislocation nucleation site. This is consistent with the LADIA strain analysis that shows that the lattice strain near the dislocation nucleation site is relatively higher in comparison with the inside of the crystal, due to the stress concentration around the surface step. We note that the average value for the area outside the white box is the same as that for the inner the crystal; however, the standard deviation of former measurement (0.18 Å) is higher than that (0.06 Å) in the later one, which is likely caused by the presence of free surfaces. Similarly, the lattice dilation in Figure 4c is characterized by measuring the distance between two neighbouring atoms along the [1̄1̄2] direction. The average values on the surface where twinning partials were emitted (white-boxed area in Supplementary Fig. S9a ); the area outside the white box and inside of the nanocrystal are: 2.75 Å (standard deviation of 0.064 Å; Supplementary Fig. S9b ), 2.52 Å (standard deviation of 0.048 Å; Supplementary Fig. S9c ) and 2.72 Å (standard deviation of 0.054 Å; Supplementary Fig. S9d ). For an unstrained lattice constant of 4.07 Å, the distance between atomic columns in the 〈112〉 direction is 2.5 Å. Identification of different dislocation types based on HRTEM images All the defects identified in our paper are based on atomic-scale lattice images. In these lattice images, each atomic column is directly imaged. Thus, any irregularity or defect in the lattice is visualized directly. Supplementary Figure S3 shows one example of how to identify a perfect dislocation ( Supplementary Fig. S3b ), a stacking fault ( Supplementary Fig. S3c ) and a twin boundary ( Supplementary Fig. S3d ) in a FCC crystal ( Supplementary Fig. S3a ). The detailed analysis procedures are described below. Perfect dislocation: A FCC unit cell is shown in Supplementary Figure S3a . If the viewing direction is [1̄10] (pointed out by a blue arrow), the atoms are projected in the [1̄10] plane, as outlined in yellow lines. In Supplementary Figure S3b , a real HRTEM lattice image of a copper crystal viewed along [1̄10] direction, showing clearly that there is an extra lattice plane in the upper part of the crystal, corresponds to a perfect edge dislocation, with its core being marked by an inverted 'T'. The Burgers vector b (marked by a light blue arrow) of this dislocation can be determined by drawing a Burgers circuit (light blue lines). The yellow, blue and pink dots correspond to the yellow, blue and pink atoms in Supplementary Figure S3a , respectively. Stacking fault: An image of the stacking fault that forms during the plastic deformation in Au nanocrystal is presented in Supplementary Figure S3c . In this image, the stacking sequences of each {111} plane are directly visualized, offering the opportunity to identify any atomic-scale stacking irregularity. It can be clearly seen that the FCC stacking sequence alters to HCP stacking order in the area pointed out by a two arrowheads and two letters 'SF', which represent stacking fault. Twinning: The upper and lower crystal in Supplementary Figure S3d show mirror symmetry, which corresponds to a twin in a FCC crystal. These results demonstrate that crystalline defects, such as perfect dislocations, partial dislocations or stacking faults and twins can be identified unambiguously based on HRTEM image. For clarity, the stacking faults can be seen more clearly in the Fourier-filtered image, as shown in Supplementary Figure S4b . In this image, the stacking of each {111} plane is clearly visible and the local hexagonal stacking can be identified (see arrowheads). Furthermore, a schematic illustration of the process shown in Figure 1a,b is plotted in Supplementary Figure S5a,b : the stacking fault is formed by the emission of the leading partial from the surface step, which is subsequently erased by the nucleation and propagation of the trailing partial dislocation. How to cite this article: Zheng, H. et al . Discrete plasticity in sub-ten-nm-sized gold crystals. Nat. Commun. 1:144 doi: 10.1038/ncomms1149 (2010).